The evolutionary origin of human hyper-cooperation Proactive, that is, unsolicited, prosociality is a key component of our hyper-cooperation, which in turn has enabled the emergence of various uniquely human traits, including complex cognition, morality and cumulative culture and technology. However, the evolutionary foundation of the human prosocial sentiment remains poorly understood, largely because primate data from numerous, often incommensurable testing paradigms do not provide an adequate basis for formal tests of the various functional hypotheses. We therefore present the results of standardized prosociality experiments in 24 groups of 15 primate species, including humans. Extensive allomaternal care is by far the best predictor of interspecific variation in proactive prosociality. Proactive prosocial motivations therefore systematically arise whenever selection favours the evolution of cooperative breeding. Because the human data fit this general primate pattern, the adoption of cooperative breeding by our hominin ancestors also provides the most parsimonious explanation for the origin of human hyper-cooperation. Compared with other primates, including the other great apes, humans show extremely intensive cooperation, which is increasingly recognized as being ultimately responsible for our unusual cognition, technology and culture [1] , [2] , [3] . A variety of mechanisms underlie this unusual level of cooperation. High social tolerance and reactive prosociality, as shown in empathy-based targeted helping where individuals respond to signs and signals of need by others, are clearly important [4] . But since these may also be found in other great apes [5] , [6] , they are evidently not sufficient to support human-like cooperativeness. Some have instead argued that a proactively prosocial motivation, also called other-regarding preference, is the critical mechanism enabling human cooperation [3] . In proactive prosociality, individuals spontaneously assist others, for instance by provisioning, without direct gains for themselves and without being solicited. Recent years have seen a growing number of studies assessing proactive prosociality in nonhuman primates. Taken together, these studies [5] , [6] revealed its presence in some nonhuman species, but not in our closest living relatives, the other great apes. The patchy distribution of proactive prosociality across species is suggestive of convergent evolution, raising the question whether the prevalence of proactive prosociality across primate species can be attributed to a particular socioecological factor. If this conjecture is confirmed, the same explanation could also account for the evolution of human proactive prosociality, and we would not need uniquely human evolutionary mechanisms, such as cultural evolution or gene-culture coevolution [2] , [3] to explain its origins in our species. Various hypotheses have been put forward to explain interspecific variation in proactive prosociality, including that it is contingent on high cognitive ability [7] , [8] , high social tolerance [9] , the need to coordinate behaviour in the context of foraging [1] , [10] , [11] , strong social bonds or allomaternal care [7] , [12] , [13] , [14] . So far, however, it has been impossible to test these hypotheses because the available data lack comparability [5] , for three main reasons. First, in humans, sharing, helping and comforting follow distinct developmental trajectories [15] and are regulated by different neural mechanisms [16] . Hence, these different mechanisms may have independent evolutionary histories. The various paradigms used to assess prosocial behaviour in nonhuman primate species may therefore have tested for different kinds of prosocial behaviour [17] , [18] , such as for reactive prosociality in targeted helping tasks and proactive prosociality in dyadic provisioning games, in which individuals can opt to provide food to a partner at no or some small cost. Since the focus here is on proactive prosociality, only a subset of prosociality studies, covering a small number of species, would be available to test the various functional hypotheses. Second, it has become evident that prosociality studies are highly susceptible to seemingly trivial methodological differences [6] , even within a single paradigm. Recent reviews have shown that some widely used dyadic provisioning games to assess proactive prosociality can yield markedly different outcomes due to small differences in payoff distributions [19] or payoff representations (for example, tokens versus real rewards [7] , [20] , [21] ). Third, studies differ with regard to whether dyads were preselected according to specific criteria, to make it more likely to detect prosocial behaviour in a species [22] , [23] . While such procedures are valid in studies aiming at a proof-of-principle, they hamper quantitative comparisons across studies and thus across species. Thus, despite a large number of prosociality studies produced over the last years, it remains difficult to distinguish true species differences from differences that result from methodological heterogeneity of the respective studies [5] , [6] . To identify the evolutionary forces that may drive proactive prosociality, we first measured proactive prosociality in a large number of species with a strictly standardized and previously validated experimental design [24] . In this group service paradigm, individuals are tested in their social group and can provide fellow group members with food without obtaining any food for themselves. We applied this test to 24 social groups of 15 primate species, ranging from lemurs (two species) to New World monkeys (seven species), Old World monkeys (two species) and apes (four species, including Homo sapiens ). In a second step, we examined correlated evolution between proactive prosociality and several socioecological factors hypothesized to contribute to variation in this trait. To disentangle the explanatory value of all the hypothesized factors, we used phylogenetic linear regressions models to control for phylogenetic non-independence of the species values, and an information-theoretic approach to model selection. To establish the general primate pattern, we initially analysed the impact of each of the potentially relevant factors in a data set that only contained nonhuman species. We then added the data on humans to test whether our species fits the general primate pattern. According to the first hypothesis, proactive prosociality is cognitively demanding and thus constrained by cognitive abilities, in particular those related to Theory of Mind reasoning [7] , [8] . As a proxy for cognitive ability, we included overall brain size in the analyses, as it is tightly linked to various measures of cognitive performance in nonhuman primates [25] . Alternatively, proactive prosociality may be cognitively demanding because it requires inhibitory control to suppress the pre-potent tendency to consume the food oneself. The presence of fission–fusion dynamics in social organization has previously been identified as an important convergent factor for the evolution of inhibitory control [26] , and was thus also included in our analyses. Second, variation in proactive prosociality among primates may be linked to social tolerance. According to the self-domestication hypothesis [9] , prosocial behaviour arises as a correlated by-product of natural selection for increased tolerance and against aggression. We therefore also assessed social tolerance in each group and included it in our analyses. Third, the need to coordinate behaviour in the context of foraging has been argued to drive proactive prosociality [1] , [10] , [11] . Among nonhuman primates, the highest coordination in foraging activity occurs in cooperative hunting. We therefore also included the presence of cooperative hunting as an explanatory variable in our models. Fourth, prosociality may be most prevalent among partners with strong social bonds. The strength of social bonds varies among primate species, and also whether they occur predominantly among males [27] , among females [28] or in mated pairs. These strong bonds are typically accompanied by cooperation, which may produce species differences in proactive prosociality. We therefore included these various types of social bonds as factors in our analyses. Because within a species, prosociality may only be expressed within the respective bond classes, we also examined intraspecific patterns and analysed in the relevant species whether proactive prosociality was over-represented in male–male dyads, female–female dyads or pair mates. Fifth, the cooperative breeding hypothesis predicts that proactive prosociality is linked to the amount of allomaternal care (care by non-mothers) provided to offspring [7] , [12] , [13] , [14] . For cooperative breeding to work, caretakers must proactively seek opportunities to provide food or other forms of help [12] . Indeed, within nonhuman primates, systematic proactive food sharing only occurs naturalistically in cooperatively breeding callitrichid monkeys, who also show the highest levels of allomaternal care [18] . We estimated the extent of allomaternal care through an updated version of a previously developed allocare score [29] , which was highly correlated with various other ways of quantifying allomaternal care. Our results demonstrate that the extent of allomaternal care provides the best explanation for the distribution of proactive prosociality among primate species, including humans. This conclusion is not affected when using different ways of quantifying allomaternal care. Importantly, we find no support for any of the other hypotheses, even when more refined analyses of within-species, dyad-level variation are conducted. The adoption of extensive allomaternal care by our hominin ancestors thus provides the most parsimonious explanation for the origin of human hyper-cooperation. Reliabilities We assessed the inter-rater reliabilities by a rater who was not the experimenter of the respective group, for 10% of all of the 389 test sessions, which included 50% of all videos of test sessions 4 and 5 of phase IV, on which the main analyses were based. The reliabilities for the transfers ranged between Cohen’s Kappa=0.89 and 1 per test session, with an average of 0.99 (s.d.=0.03); the reliabilities for the reaching data ranged between 0.67 and 0.83 (average=0.75, s.d.=0.07). All analyses were based on the data from the first rater. 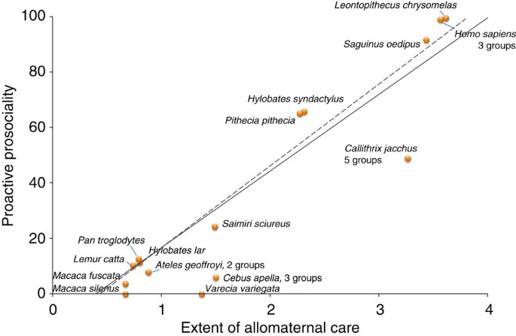Figure 1: Proactive prosociality as a function of the extent of allomaternal care in a sample of 15 primate species. Solid regression line: excludingHomo sapiens; dotted regression line: includingHomo sapiens. Proactive prosociality refers to the percentage of trials with food transfers to other group members during the last two test sessions in phase IV of the experiment, by individuals passing control criterion 1. Between-species variation in proactive prosociality In nonhuman primates, among the various potential factors ( Supplementary Tables 1–3 ), allomaternal care emerged as the best predictor in unifactorial analyses of the interspecific variation in proactive prosociality ( Table 1 , Fig. 1 ), along with weakly significant effects of social tolerance and pair bonds (both positive) and brain size (negative; Fig. 2 ). Moreover, in all models containing a combination of any two of these factors, as well as their interactions, allomaternal care emerged as the only significant effect on proactive prosociality, whereas none of the interaction effects were significant ( Supplementary Table 4 ). The best-fitting model, chosen according to the lowest value of the Akaike Information Criterion corrected for small sample size, included allomaternal care only ( Fig. 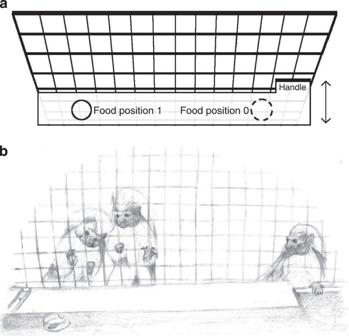Figure 4: Group service apparatus. (a) Schematic drawing. The board with the food bowl in position 0 or 1 is attached outside the wire mesh of the home cage. Subjects can pull the handle to move the board to within reach (as indicated by the grey arrow), but the board slides back if the subject releases the handle. Subjects can pull the board and retrieve the food themselves if the food bowl in position 0 is baited. However, food baited in position 1 can only be made available if one individual pulls the handle and holds the board within reach, while a second individual retrieves the food. (b) A cotton-top tamarin (Saguinus oedipus) pulls the board to provide food in the transparent bowl to other group members. Line drawing after still frame. 1 , Table 1 ). Table 1 Comparative tests of the hypotheses for the evolution of proactive prosociality. Full size table Figure 1: Proactive prosociality as a function of the extent of allomaternal care in a sample of 15 primate species. Solid regression line: excluding Homo sapiens ; dotted regression line: including Homo sapiens . 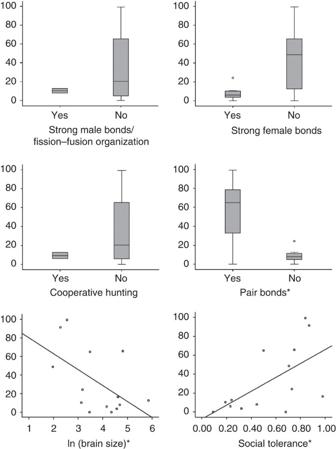Proactive prosociality refers to the percentage of trials with food transfers to other group members during the last two test sessions in phase IV of the experiment, by individuals passing control criterion 1. Figure 2: Proactive prosociality as a function of the explanatory variables other than the extent of allomaternal care (withoutHomo sapiens). The presence (n=2) or absence (n=12) of strong male bonds or fission–fusion organization in a species, of strong female bonds (present in five species, absent in nine), of cooperative hunting (present in two species, absent in 12), of pair bonds (present in seven species, absent in seven) as well as brain size and social tolerance. The box plots represent medians (black horizontal lines), inter-quartile range (grey boxes), minima and maxima (whiskers) as well as outliers (dots) *P<0.05. Full size image Figure 2: Proactive prosociality as a function of the explanatory variables other than the extent of allomaternal care (without Homo sapiens ). The presence ( n =2) or absence ( n =12) of strong male bonds or fission–fusion organization in a species, of strong female bonds (present in five species, absent in nine), of cooperative hunting (present in two species, absent in 12), of pair bonds (present in seven species, absent in seven) as well as brain size and social tolerance. The box plots represent medians (black horizontal lines), inter-quartile range (grey boxes), minima and maxima (whiskers) as well as outliers (dots) * P <0.05. Full size image In the next step, we repeated the same analyses after adding the results from the human subjects (three groups of 4:5–7:1-year-old Kindergarten children) into the nonhuman primate data set. As in the previous data set, the best model only included allomaternal care. Unifactorial effects were again present for social tolerance and pair bonds, but lost most of their explanatory power in two-factorial models that also included allomaternal care ( Supplementary Table 5 ). To assess how well the human data fit the general primate pattern, we also calculated the standardized residuals for all species (mean=0, s.d.=1), including humans, relative to the regression line based on nonhuman primates only. Humans deviated from this regression line by less than one s.d. (0.85), indicating that they do not represent an outlier and therefore follow the general primate pattern. Thus, allomaternal care provides the best explanation for the distribution of proactive prosociality among primate species, including humans. Importantly, these results are robust to different ways of quantifying allomaternal care ( Supplementary Table 6 ). Dyad-level variation in proactive prosociality Because some of these alternative hypotheses also make predictions regarding variation within the groups, more refined tests of dyad-level patterns are also possible. First, if proactive prosociality is linked to male bonding, we expect more transfers between male–male dyads in male-bonded species (spider monkeys: Ateles geoffroyi ; chimpanzees: Pan troglodytes ) than between other types of dyads. However, in test sessions 4 and 5 of phase IV, in both species transfers between male–male dyads did not occur more than expected ( Fig. 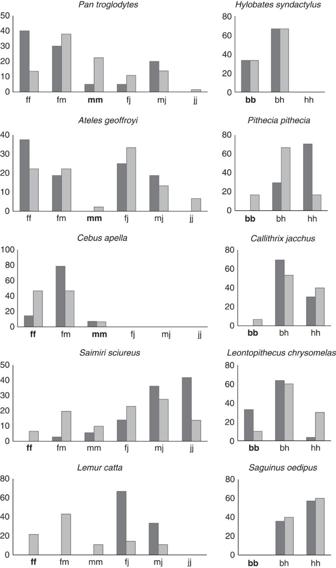3 ; chimpanzees: χ 2 =2.48, df=1, ns; spider monkeys: absolute number of transfers too low to allow for statistical testing), and the pattern of within-group variation is thus consistent with the rejection of the male bonding hypothesis. Figure 3: Distribution of transfers per dyad type. Dyad types printed in bold are expected to be over-represented by different alternative hypotheses, that is, in male–male dyads (mm) in species with strong male bonding and/or cooperative hunting, in female–female dyads in species with strong female bonding or in mate pairs in pair-bonded species.Xaxis: dyad type,yaxis: % of transfers in sessions 4 and 5 of phase IV. Light-grey bars represent expected values, dark-grey bars observed values. b, breeder; f, adult female; j, juvenile; h, offspring of breeding pair, that is, helpers; m, adult male.Pan troglodytes: 55 female–female dyads (55ff), 154fm, 91mm, 44fj, 56mj, 6jj;Ateles geoffroyi: 10ff, 10fm, 1mm, 15fj, 6mj, 3jj;Cebus apella: 21ff, 21fm, 3mm;Saimiri sciureus: 10ff, 30fm, 15mm, 20fj, 24mj, 6jj;Lemur catta: 1ff, 6fm, 3mm, 6fj, 9mj;Hylobates syndactylus: 1bb, 2bh;Pithecia pithecia: 1bb, 4bh, 1hh;Callithrix jacchus(Jojoba): 1bb, 8bh, 6hh;Leontopithecus chrysomelas: 1bb, 6bh, 3hh;Saguinus oedipus: 0bb, 4bh, 6hh). Figure 3: Distribution of transfers per dyad type. Dyad types printed in bold are expected to be over-represented by different alternative hypotheses, that is, in male–male dyads (mm) in species with strong male bonding and/or cooperative hunting, in female–female dyads in species with strong female bonding or in mate pairs in pair-bonded species. X axis: dyad type, y axis: % of transfers in sessions 4 and 5 of phase IV. Light-grey bars represent expected values, dark-grey bars observed values. b, breeder; f, adult female; j, juvenile; h, offspring of breeding pair, that is, helpers; m, adult male. Pan troglodytes : 55 female–female dyads (55ff), 154fm, 91mm, 44fj, 56mj, 6jj; Ateles geoffroyi : 10ff, 10fm, 1mm, 15fj, 6mj, 3jj; Cebus apella : 21ff, 21fm, 3mm; Saimiri sciureus : 10ff, 30fm, 15mm, 20fj, 24mj, 6jj; Lemur catta : 1ff, 6fm, 3mm, 6fj, 9mj; Hylobates syndactylus : 1bb, 2bh; Pithecia pithecia : 1bb, 4bh, 1hh; Callithrix jacchus (Jojoba): 1bb, 8bh, 6hh; Leontopithecus chrysomelas : 1bb, 6bh, 3hh; Saguinus oedipus : 0bb, 4bh, 6hh). Full size image Second, the same prediction of a male bias in transfers results from the cooperative hunting hypothesis, because group hunting is predominantly biased towards males, both in chimpanzees and capuchin monkeys [27] . However, in both species, transfers are not biased towards male–male dyads ( Fig. 3 : capuchin monkeys: absolute number of transfers too low to allow for statistical testing), which is inconsistent with the cooperative hunting hypothesis. Third, if female bonding determined the variation in proactive prosociality, we would expect a bias towards female–female dyads among the female-bonded species (macaques: Macaca fuscata , Macaca silenus ; squirrel monkeys: Saimiri sciureus ; ring-tailed lemurs: Lemur catta ; capuchin monkeys: Cebus apella ). Overall, transfers were rare in these species and did not allow for statistical testing; nevertheless, the transfers that did happen were not biased towards female–female dyads ( Fig. 3 for squirrel monkeys, capuchin monkeys and ring-tailed lemurs). In Macaca silenus , no transfers occurred in sessions 4 and 5; in Macaca fuscata , only seven transfers occurred, and in six of these, the juvenile daughter of the dominant female was involved. Taken together, the within-group variation in female-bonded species thus confirms the rejection of the female bonding hypothesis. Finally, if pair bonding were an important independent determinant of proactive prosociality, we would expect most transfers to occur between pair mates. Although pulling was non-random between dyad types in the sakis ( Pithecia pithecia : χ 2 =15.6, df=1, P <0.001), the male never pulled for anybody and transfers between the pair mates were absent. In the gibbons ( Hylobates lar ), we could not test this prediction because the breeding pair could only pull for each other (the infant was too young to pull or take food). In the siamang ( Hylobates syndactylus ) group, composed of the breeding pair and a juvenile son, transfers were not more likely between the pair mates ( χ 2 =0, df=1, nonsignificant) and all transfers were initiated either by the father (33.3%) or the son (66.6%). In the ruffed lemurs ( Varecia variegata ), no transfers occurred in test session 4 and 5. In common marmosets, transfers were also not biased towards the breeding pair but instead occurred less than expected by chance ( χ 2 =8.5, df=1, P =0.004). In cotton-top tamarins ( Saguinus oedipus ), the breeding female had died, so no test was possible. Overall, then, no bias towards more transfers within the pair bond was apparent. The only exception was encountered in the lion tamarins ( Leontopithecus chrysomelas ), where transfers were more likely between breeders than between other dyads ( χ 2 =81.27, df=1, P <0.001). However, in this group, 37.5% of the food rewards made available through pulling within the breeding pair were further shared with an infant, and food sharing was presumably constrained by increasing satiation of the immature over the 70 test trials, rather than by a lack of willingness to share. This pattern does not support the idea that pair mates exclusively pulled for each other. Furthermore, when we removed the breeding female from the group for an additional test session with the remaining group members, this did not appreciably decrease the overall number of transfers compared to the last regular test session (98.6% in the last regular test session, compared to 90.0% in the additional test session without the breeding female). Taken together, these within-group findings do not support pair bonding as the sole determinant of proactive prosociality. The within-species, dyad-level analyses therefore likewise did not provide support for any of the bonding hypotheses, corroborating the result of the species-level analyses. The results of the between-species comparative analyses suggest that allomaternal care best predicts proactive prosociality in primates. This finding is corroborated by the results of the within-species tests of dyadic patterns (see Supplementary Discussions for details) and unlikely to be based on a methodological artefact (see Supplementary Methods for details). While the group service paradigm deployed here is simple and robust, it has two limitations as compared with the usual tests involving separated dyads. First, its statistical power is limited, because groups (or even species) rather than individuals represent independent data points. However, group testing ensures greater ecological validity than dyadic tests because it assesses the behaviour of individuals in their naturalistic context, rather than after separation from the rest of the group; ecological validity is crucial to testing functional hypotheses. A second weakness, which it shares with other prosociality tests, is that it may be sensitive to minor methodological changes (for example, size of the apparatus or time of testing relative to last feeding). However, these factors do not systematically covary with species in the present data set. In fact, we explicitly controlled for such potential effects by standardizing the methods across groups and species through the use of identical protocols and experimental setups. Whether changes in the protocol or experimental setup indeed influence performance in the group service paradigm, and in what way, remains to be established in future studies. A more general limitation of our approach is that we used only a single test for the proactively prosocial motivation, whereas convergent results of multiple tests would enhance confidence in our findings. Thus, the development of a robust standardized dyadic test, and its systematic application to multiple species, to complement the group service approach, continues to have a high priority. Such dyadic tests would also provide an important complement to the tests of within-group patterns of proactive prosociality across species applied in the group service paradigm. Nonetheless, the various controls applied in the present study indicate that it is unlikely that any artefact or systematic bias is responsible for the strong pattern obtained here. For a more thorough discussion of how the present results link to earlier prosociality studies, see Supplementary Discussion . Having established that the result obtained here is likely to survive additional testing, we can now address its implications. Unlike any of the other apes, humans have become cooperative breeders, perhaps in response to moving into savannah habitats, where immature foraging success was severely impaired [14] , [30] . The pattern reported here therefore supports an evolutionary scenario in which the adoption of shared childcare by our ancestors modified our prosociality, by convergently adding a proactive motivation, as is the rule in other primate lineages that adopt cooperative breeding. This motivation may have transformed the individualistic cognitive skills as present in great apes (but not in monkeys) into the human-typical shared intentionality [1] , which in turn produced cascading cognitive effects via language, collaboration and instructed learning [10] . These results therefore support the cooperative breeding hypothesis [12] , [13] , [14] for the evolution of this critical element of human hyper-cooperation. A major feature of this hypothesis is that it explains why only our hominin ancestors, and none of the other, independently breeding great apes, took this extraordinary evolutionary trajectory [14] . This hypothesis can also explain why our hyper-cooperation also extends to non-kin. First, obligate cooperative breeders usually contain mostly kin, that is, offspring of the unrelated breeding pair, but when unrelated individuals join these groups, their behaviour is often indistinguishable from that of the related helpers [22] , [31] , [32] . Second, human forager groups contain multiple mated pairs, and obligations towards the mate’s relatives, which genetically speaking are non-relatives, are also important. Thus, once established in our ancestors, the proactively prosocial psychology may have become generalized toward all in-group members [33] . Finally, this general biological explanation for the origin of human hyper-cooperation also helps delineating the contexts in which uniquely human evolutionary processes relying on cultural evolution, group selection, cultural group selection or gene-culture coevolution [1] , [2] , [3] are needed to bring about human hyper-cooperation. Since in small face-to-face groups, hyper-cooperation works well without additional mechanisms such as altruistic punishment [2] , [3] , it is likely that these processes only became necessary to maintain hyper-cooperation in large, anonymous societies, but were not needed earlier. Subjects Table 2 provides an overview of the subjects that participated in the experiment. In various institutions, we tested all subjects in their social group, in their home cage in between the regular feedings. The animals were neither food- nor water-deprived. As rewards, we used special treats that were highly preferred by all group members, as established before the test. Immatures too small to handle the apparatus or take food through the wire mesh were omitted in measures of social tolerance and whenever the analysis involved calculation of expected values. Other individuals who had not reached sexual maturity at the beginning of the test were included and classified as juveniles. Table 2 Origin and composition of the social groups tested with group service. Full size table The human children were tested in their Kindergarten groups, in a separate room but in the same building as their classroom. To minimize the possibility that socially desired behaviour would be elicited by the presence of an authority figure, we tested human children in the absence of teachers (see also Supplementary Methods for further details on testing human children, and Supplementary Fig. 1 ).The experiments with the nonhuman primates had been approved by the relevant authorities; those in Zurich and Basel by the Kantonales Veterinäramt, under the license numbers 4389 and 2541, respectively. For the human children, the parents gave written informed consent for their children’s participation, and the study was approved by the Ethik-Kommission of the Kinderspital Zurich, Unterkommission SPUK. The group service paradigm We used an approach explicitly developed to provide a standardized measure of both proactive prosociality and social tolerance, the group service paradigm [24] . In essence, social groups are presented with food that is out of reach, on a board outside their home cage ( Fig. 4 ). By pulling the handle of the board, an individual can pull food within reach of other group members. However, the pulling individual can never obtain the food for itself, because (i) the food is too far away from the handle to both pull and simultaneously retrieve the food and (ii) the board slides back automatically as soon as the handle is released. The only way for any group member to obtain food is when some other individual pulls the handle and holds it long enough for the group member to retrieve the food from the board. The group service experiment consists of five phases, and subjects have to pass predefined criteria to enter the subsequent phases. Various control conditions and criteria are an integral part of the group service approach to ensure that the behaviour indeed qualifies as proactive prosociality [24] . Figure 4: Group service apparatus. ( a ) Schematic drawing. The board with the food bowl in position 0 or 1 is attached outside the wire mesh of the home cage. Subjects can pull the handle to move the board to within reach (as indicated by the grey arrow), but the board slides back if the subject releases the handle. Subjects can pull the board and retrieve the food themselves if the food bowl in position 0 is baited. However, food baited in position 1 can only be made available if one individual pulls the handle and holds the board within reach, while a second individual retrieves the food. ( b ) A cotton-top tamarin ( Saguinus oedipus ) pulls the board to provide food in the transparent bowl to other group members. Line drawing after still frame. Full size image The group service paradigm provides comparable data due to the standardization of the experimental procedure, but also has additional advantages. First, the setup is cognitively non-demanding, and even small-brained primate species, like callitrichid monkeys, can demonstrably understand it and pass all necessary control conditions [24] . Second, the test does not require that individuals be separated from their group mates, which may especially affect performance in highly interdependent species. Third, the test quantitatively assesses the degree of proactive prosociality as it occurs in a naturalistic situation, rather than in specific dyads or under specific circumstances. Fourth, phase II of the group service paradigm also provides a repeatable measure of social tolerance in the group concerned. Apparatus and procedure The apparatus consisted of a board placed outside the wire mesh of the home cage. A food bowl could be placed on top of the board ( Fig. 4 ). If it was placed in position 0, a subject could pull the handle with one hand and access the food with the other hand. However, if the bowl was placed in position 1, which was always located more than two arms’ lengths away from position 0, the subject pulling the handle was no longer able to access the bowl by herself. Position 0 was used in training and motivation trials, position 1 in test trials. Importantly, the board was mounted on inclined rails that ran perpendicular to the mesh, so that the board would slide down away from the cage unless it was pulled by the handle. Only if it was pulled by one individual and held in place close to the wire mesh would its content become accessible to the remaining subjects in the home cage. Successful food provisioning in the group service test thus required that one individual left the position closest to the food, moved to the position in front of the handle and pulled and held it in a way that was sufficiently coordinated to allow a second individual to retrieve the food. The group service test was composed of five distinct experimental phases, and subjects had to pass predefined criteria to enter the subsequent phase. Phase I, Habituation—The aim of phase I was to habituate the subjects to the apparatus, the basic procedure and the experimenter. The board with the food bowl in position 0 was fixed close to the wire mesh so that subjects could freely access the bowl without having to pull the apparatus. Pieces of favourite foods (minimum 10 pieces per subject) were provided sequentially in position 0 during 5 days, or until every subject had taken at least three pieces. In each trial, a piece of food was held up by the experimenter who drew the subjects’ attention to it verbally by saying: ‘look here’! This attention-getting procedure assured that all subjects of a group would pay attention to the setting, independent of cage size, and was used in all phases of the experiment. If necessary, dominant individuals were distracted from the apparatus by a second experimenter to make sure that all individuals would approach the apparatus. Phase II, Social tolerance—In phase II, we quantified social tolerance in the feeding context, by placing 35 pieces of favourite food, one at a time, on the apparatus fixed within reaching distance of the subjects, as in phase I. When a piece of food was taken by an individual, we waited until the food was completely consumed before starting the next trial by saying ‘look here!’ and placing the next piece of food in the bowl. We recorded the percentage of food items received by each group member and calculated the evenness J' of this distribution [34] , as a measure of how equitable food was obtained by group members, and thus, how good the odds of subordinates were of having access to the food. When food was shared (passively or actively), it was counted as food received by both group members involved, independently of the amount of food eaten by each individual. To assess the repeatability of this measure of social tolerance, we conducted this test twice, on two consecutive days. Across the 24 primate groups, the evenness of the distribution on day one was strongly correlated with that on day two ( r 2 =0.722, P <0.001), which provides evidence for high repeatability of this measure of social tolerance. For the main analyses, we calculated the amount of social tolerance of each group based on the combined data of both days. Phase III, Training—In phase III, the subjects learned to pull the handle and hold it to retrieve the food. The board was now in its original position, at some distance from the wire mesh, such that only the handle could be reached. Criterion was reached when the subjects were able to pull the handle, hold it with one hand and take food with the second hand, with the food bowl placed within one arm’s length from the handle ( Fig. 4 , position 0). Pieces of food were provided until each subject passed the criterion of pulling the food within reach for itself in at least seven trials (again, if necessary after distracting dominant individuals). For individuals who had difficulties in learning the task, we added intermediate steps, such as placing the food on top of the handle, directly in front of the handle, near the handle with increasing distances to it and finally in the food bowl. Passing the criterion of phase III corresponds to passing the knowledge probe that individuals did understand how the apparatus worked. Phase IV, Group service—In phase IV, the core of the group service experiment, we measured proactive prosociality. The board was in its original position as in phase III, but food was now placed in position 1, too far away for an individual to pull the board and at the same time retrieve the food for itself. Essentially, we assessed how much food each group was able to make available to its members, which required individuals to forgo the reward for themselves and instead move away from the food to pull and hold the handle and provide the food to its group mates. In phase IV, we alternately ran five test sessions and five control sessions. Each session consisted of 70 regular and 14 motivation trials. During regular trials, food was placed in position 1 and could only become available to the group if an individual would forgo the reward and instead pull for its group members. During motivation trials, food was placed in position 0 and could be obtained by individual effort (like in Phase III). Motivation trials were inserted after every 5th regular trial, resulting in a total of 84 trials, including the very first trial, which was also a motivation trial. Motivation trials, which included the vocal attention getters, were included to assess whether the animals were interested in the reward until the end of each test, and would continue to attend to the experimental setup. If no one would take the food in more than two consecutive motivation trials in less than 1 min, the experimenter ended the session. In the majority of groups, all motivation trials were always taken, both in test and control sessions (exceptions where food was not taken in two consecutive motivation trials at least once over the five test and five control sessions: siamangs, one group of spider monkeys, lemurs and kattas). During test sessions, the food bowl was baited at the beginning of each trial by holding up the food item, attracting the group’s attention by a vocal attention getter (‘look here!’) and conspicuously placing the food item in the bowl. The trial ended either when the food had been provided to a group member or after 1 min had elapsed. If no food was taken in a trial, the experimenter started the next trial by holding up the food item from the bowl again, showing it demonstratively to the group, attracting their attention vocally and placing it back in the food bowl. During control sessions, the food bowls were not baited with food in regular trials. Instead, the experimenter held up a small stick, touched the bowl with it audibly and simultaneously used the same verbal attention getter as during the experimental trials. This control served to exclude the possibility that pulling occurred simply to explore the apparatus itself, or as mere play behaviour. As in the test sessions, motivation trials, in which real food was provided, were inserted after every 5th regular trial. Proactive prosociality was calculated as the corrected percentage of food provisioning in the last two test sessions for each group. The last two test sessions were chosen because by then, all subjects had had ample opportunity to learn that they could not get the food by themselves by pulling the apparatus, which in the very first trials may have led to false positives. The last two test sessions thus yield the most conservative estimate of proactive prosociality, but the results do not change if we take the total percentage of food provisioning overall test sessions. Furthermore, the percentage was corrected by including in this measure only provisioning by individuals who passed the criterion of pulling significantly more in test versus control sessions, but note that both measures are highly correlated ( Supplementary Fig. 2 ). Phase V, excluding alternative explanations for sustained provisioning—If sustained provisioning occurred over the five test sessions in phase IV, it could still be that transfers occurred by mistake because the pulling subjects had not understood that they wouldn't be able to obtain the food themselves, and had not learnt this during the five test sessions. Even though the animals would have had numerous opportunities to learn that pulling food in position 1 was never rewarded, it could be argued, especially for smaller-brained species such as callitrichids that 350 trials are not sufficient to learn so. In the final phase V, we therefore tested this understanding, but obviously could only do so in those groups that had shown sustained provisioning in phase IV, that is, who continued to provide food to partners at stable rates throughout the 5 test sessions of phase IV. Phase V was identical to phase IV, except that physical access to the food bowl was now blocked by a fine-meshed grid attached to the home cage in front of position 1, leaving visual and olfactory cues present. Thus, even if the tray was pulled to within reach, no one could ever obtain the food. In the sakis and in one group of common marmosets, instead of blocking the access with a fine-meshed grid, we moved the apparatus to the edge of the cage so that the outer part of the apparatus would overhang the length of the home cage. Thus, the apparatus could still be pulled but the food would nevertheless not become available to the other group members. We again ran five test sessions (position 1 baited) and five control sessions (position 1 empty) with the grid always in place, on alternating days. Each session consisted of 70 trials and additional motivation trials interspersed after every 5th regular trial (during motivation trials, food was again available and accessible in position 0). If in phase IV, pulling the baited tray in position 1 occurred for any reason other than intentionally providing food (for example, a persistent inability to inhibit pulling the baited tray due to the salient visual and olfactory cues), pulling should continue in phase V at the same level as during phase IV. However, if pulling in phase IV occurred to provide food to group members, pulling in phase V should decrease over time more consistently than in phase IV because pulling in phase V did not result in providing food to group members. Data coding and reliabilities All sessions in phase III, IV and V were video recorded. During the experiments, data were also collected by hand, including whether an individual pulled or not within a given trial, whether a transfer occurred and if so, the identity of the donor and the recipient. This data was later verified with the video clips by the experimenter. In case of inconsistencies, the true values based on the video clips were used. Reaching was only coded from the videos after the experiment, for test session 5 of phase IV. For each regular trial, we coded whether an individual tried to reach for the food in position 1 by extending its arm (or tail in the case of spider monkeys) outside of the wire mesh in the direction of the food reward. However, we only included reaching attempts that could be perceived by a second individual that was close enough to reach the apparatus with one leap (exact distances differed according to the respective species). Validity of the group service approach The group service paradigm requires several criteria to be fulfilled to conclude that food deliveries are due to proactive prosociality [24] (see Supplementary Methods for details). First, subjects must understand the task. They must pass various knowledge probes and control conditions to proceed to the experiment ( Supplementary Table 7 ). In particular, the results must not reflect the absence of sufficient inhibitory control. Ideally, an alternative measure that controls for inhibitory control (that is, difference scores for which pulling rates during control sessions are subtracted from pulling during test sessions, Supplementary Table 8 ) produces the same results as those obtained with the absolute measure used for the main analyses. Second, species with high rates of proactively prosocial pulling must maintain high rates throughout all five test sessions, and not decline over time, as would be expected if animals unintentionally provisioned others in the beginning and gradually learned they were doing so ( Supplementary Fig. 3 ). Third, we must exclude that reactive prosociality drives the results, that is, that begging is not necessary and other signs of need by recipients ineffective ( Supplementary Fig. 4 ). Fourth, phase V is added to further demonstrate the understanding of the consequences of their pulling. However, this is only necessary for those groups passing the three criteria mentioned above and continuing to provide food in more than 40% of all trials in the last test session. Note that for the human children, phase V was modified ( Supplementary Methods and Supplementary Fig. 6 ). Finally, one could argue that rather than testing different groups, we only assess the behaviour of the most dominant individual per group because this is the only individual in the group enjoying near-complete freedom in behaviour. To test this possibility, we assessed whether the relationship between the extent of allomaternal care and proactive prosociality also holds at the group level (GLM; response: proactive prosociality, random effect: species. Note that phylogenetic structure can only be taken into account in species-level analyses. However, lambda was low or 0 in most of the species-level analyses performed in the main analyses, suggesting that phylogenetic structure has only a marginal effect in the present data set). Confirming our main conclusion, the relationship between allomaternal care and proactive prosociality is also stable when we test at the group level (F (13,10) =6.24, P =0.003, Supplementary Fig. 5 ). How to cite this article: Burkart, J. M. et al . The evolutionary origin of human hyper-cooperation. Nat. Commun. 5:4747 doi: 10.1038/ncomms5747 (2014).